Evidence of a field-induced Berezinskii–Kosterlitz–Thouless scenario in a two-dimensional spin–dimer system Two-dimensional (2D) systems with continuous symmetry lack conventional long-range order because of thermal fluctuations. Instead, as pointed out by Berezinskii, Kosterlitz and Thouless (BKT), 2D systems may exhibit so-called topological order driven by the binding of vortex–antivortex pairs. Signatures of the BKT mechanism have been observed in thin films, specially designed heterostructures, layered magnets and trapped atomic gases. Here we report on an alternative approach for studying BKT physics by using a chemically constructed multilayer magnet. The novelty of this approach is to use molecular-based pairs of spin S =½ ions, which, by the application of a magnetic field, provide a gas of magnetic excitations. On the basis of measurements of the magnetic susceptibility and specific heat on a so-designed material, combined with density functional theory and quantum Monte Carlo calculations, we conclude that these excitations have a distinct 2D character, consistent with a BKT scenario, implying the emergence of vortices and antivortices. Magnetic insulators, composed of weakly interacting pairs (dimers) of antiferromagnetically coupled S =1/2 spins, offer exciting possibilities for studying finite-temperature critical phenomena under well-controlled conditions [1] . Prominent examples include the Bose–Einstein condensation (BEC) of magnetic triplet excitations (triplons), first observed in TlCuCl 3 (refs 2 , 3 ) and subsequently in a variety of related compounds, see ref. 4 for a recent review. Besides the fascinating possibilities that coupled-dimer systems offer in exploring the behaviour of interacting quantum particles in three dimensions (3D), they also enable the studying of effects of reduced dimensionality, especially 1D behaviour [5] , and effects related to dimensional crossovers [6] , [7] , see refs 8 , 9 for a critical discussion. It is thus natural to ask whether dimers, properly combined, can also be used to explore phenomena restricted to 2D. For interacting particles in 2D, long-range magnetic order and BEC are destroyed by thermal fluctuations as was rigorously shown in ref. 10 . Instead, according to the Berezinskii, Kosterlitz and Thouless (BKT) theory, a topological order may occur resulting from the binding of vortex–antivortex pairs [11] , [12] , [13] . The BKT theory has been applied to a variety of 2D phenomena in thin films, specially designed heterogeneous systems [14] , [15] , [16] , [17] , [18] , [19] , [20] , [21] , trapped atomic gases [22] , as well as layered bulk magnets [23] , [24] , [25] , [26] , [27] , [28] . Here we report on an alternative approach for studying BKT physics. The novelty of this approach is to use molecular-based dimers as magnetic building blocks and to take advantage of synthetic chemistry to assemble these objects into layers with large inter -layer spacing. On the basis of this design strategy, we recently synthesized a metal-organic copper (spin S =1/2)-containing compound [29] , which lacks long-range 3D magnetic order down to 27 mK, the lowest temperature accessible by our experiment. By using high-resolution magnetic susceptibility and specific heat measurements, together with elaborate ab initio calculations and quantum Monte Carlo (QMC) simulations, we demonstrate that the system shows distinct 2D behaviour in its magnetic properties, implying vortices as topologically stable excitations. Material, crystal structure and magnetic exchange couplings The material is a member of a newly discovered series of coordination polymers formed by assembling Cu-based dimer-building blocks, where hydroquinone-derived linkers were used to connect the magnetic S =1/2 Cu 2+ ions in a dimer unit [29] , [30] , [31] , [32] . The moderate strength of the intra -dimer couplings of J d /k B ~10 K that can be realized by this design strategy [31] implies that a moderately strong field of several Tesla is sufficient to close the spin gap separating the lower ( S z =+1) branch of the excited triplon bands from the spin-singlet ground state. This property together with the high degree of tunability by chemical means makes these novel spin–dimer systems particularly suitable for exploring field-induced magnetic phenomena. High-quality single crystals of the complex dimer material C 36 H 48 Cu 2 F 6 N 8 O 12 S 2 (abbreviated to TK91 in the following) have been synthesized [29] . The system, crystallizing in a triclinic structure (space group ) has a layered structure where planes, containing polymeric chains along the crystallographic a axis, are separated by CF 3 SO 3 − groups, cf . Fig. 1 . Single crystal X-ray diffraction yields a high degree of crystalline perfection [29] . According to low-temperature magnetic measurements on a variety of single crystals derived from various batches, the concentration of S =1/2 impurities is usually less than 0.5% but has never exceeded 0.8%. 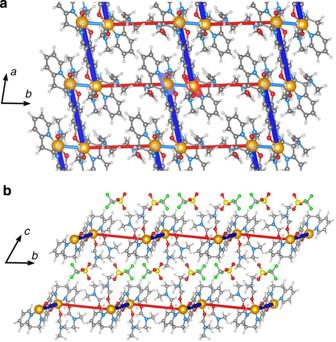Figure 1: Crystal structure and spin–spin interactions of TK91. Crystal structure, containing two Cu ions per unit cell, viewed perpendicular to theabplane (a) and perpendicular to thebcplane (b) with the main building blocks highlighted. Ina, the triflate counterions CF3SO3−are omitted for clarity. The spin (S=1/2)-carrying copper ions are shown as orange spheres. Red, blue, grey, yellow and green spheres denote oxygen, nitrogen, carbon, sulfur and fluorine atoms, respectively. The thick, dark-blue rods indicate the dominant magnetic Cu–Cu exchange interaction mediated via the modified hydroquinone group by whichS=1/2 dimers are formed. Weaker Cu–Cu interaction paths, mediated via oxygen atoms across a distanced1Cu–Cu=3.28 Å and via DMF (C3H7NO) solvent molecules across a distanced2Cu–Cu=9.301 Å are indicated by thin cyan and thin red rods, respectively. DFT total energy calculations yield for the former an exchange coupling constantJ1/kB=2.1 K. This coupling includes weak δ-bondings, indicated exemplarily by parallel blue and red planes representing the location of the Cu-dx2−y2orbitals. For the latter interaction acrossd2Cu–Cu, the calculations yieldJ2/kB=0.6 K. Panel (b) shows that theabplanes are separated by the CF3SO3−groups with Cu–Cu distances ofd3Cu–Cu=13.78 Å, corresponding toJ⊥=0 in our DFT calculations. The thermal stability of the structure was studied in ref.32. According to this work, the loss of DMF solvent molecules is accompanied by a considerable change of the magnetic properties32, which can be readily identified and thus excluded to be of relevance for the observations discussed here. Figure 1: Crystal structure and spin–spin interactions of TK91. Crystal structure, containing two Cu ions per unit cell, viewed perpendicular to the ab plane ( a ) and perpendicular to the bc plane ( b ) with the main building blocks highlighted. In a , the triflate counterions CF 3 SO 3 − are omitted for clarity. The spin ( S =1/2)-carrying copper ions are shown as orange spheres. Red, blue, grey, yellow and green spheres denote oxygen, nitrogen, carbon, sulfur and fluorine atoms, respectively. The thick, dark-blue rods indicate the dominant magnetic Cu–Cu exchange interaction mediated via the modified hydroquinone group by which S =1/2 dimers are formed. Weaker Cu–Cu interaction paths, mediated via oxygen atoms across a distance d 1 Cu–Cu =3.28 Å and via DMF (C 3 H 7 NO) solvent molecules across a distance d 2 Cu–Cu =9.301 Å are indicated by thin cyan and thin red rods, respectively. DFT total energy calculations yield for the former an exchange coupling constant J 1 / k B =2.1 K. This coupling includes weak δ-bondings, indicated exemplarily by parallel blue and red planes representing the location of the Cu- d x 2 − y 2 orbitals. For the latter interaction across d 2 Cu–Cu , the calculations yield J 2 / k B =0.6 K. Panel ( b ) shows that the ab planes are separated by the CF 3 SO 3 − groups with Cu–Cu distances of d 3 Cu–Cu =13.78 Å, corresponding to J ⊥ =0 in our DFT calculations. The thermal stability of the structure was studied in ref. 32 . According to this work, the loss of DMF solvent molecules is accompanied by a considerable change of the magnetic properties [32] , which can be readily identified and thus excluded to be of relevance for the observations discussed here. Full size image The peculiar magnetic properties of TK91 result from Cu 2+ ( S =1/2)-containing dimers (with an intra -dimer Cu–Cu distance of d Cu–Cu =8.36 Å) formed by modified hydroquinone units and their mutual interactions along the different exchange paths in the 3D crystalline network, see Fig. 1 . The dimer–dimer couplings may involve indirect Cu–Cu exchange interactions mediated via oxygen atoms ( d 1 Cu–Cu =3.28 Å), coordinated Dimethylformamide (C 3 H 7 NO) solvent molecules ( d 2 Cu–Cu =9.301 Å) as well as CF 3 SO 3 − groups ( d 3 Cu–Cu =13.78 Å). For a reliable estimate of the nature and strength of the interaction paths and in order to derive an effective Hamiltonian for describing the low-energy properties, elaborate ab initio density functional theory (DFT) calculations together with N-th order muffin tin orbital (NMTO) downfolding studies have been performed, which take into account all structural and chemical aspects appropriately. The NMTO downfolding [33] of the DFT bandstructure, which consists of deriving a low-energy Hamiltonian by the Löwdin partition method [34] , points to the presence of two largest Cu–Cu hopping parameters t d =34 meV and t 1 =12 meV followed by smaller ones (<10 meV) t 2 and t 3 . These values indicate that the Cu ions, linked by the modified hydroquinone group, have the strongest couplings and form dimers. A perturbative estimate of the antiferromagnetic contribution to the exchange constant, J d =4 t d 2 / U with U =6 eV (an appropriate value for Cu in the present coordination environment) yields an intra -dimer interaction J d / k B =8.9 K. In order to obtain accurate estimates of the Cu–Cu exchange interactions, we proceeded by mapping LSDA+ U ( U =6 eV) total energy differences of TK91 supercells with various Cu-spin configurations on a spin-1/2 Heisenberg model. We obtain J d / k B =9.4 K (in very good agreement with the perturbative estimate above), J 1 / k B =2.1 K (corresponding to Cu ions at distances d 1 Cu–Cu =3.28 Å), J 2 / k B =0.6 K ( d 2 Cu–Cu =9.301 Å) and an inter -layer coupling J ⊥ / k B ≈0 ( d 3 Cu–Cu =13.78 Å). The resulting spin–spin interaction network has the topology of a 2D distorted honeycomb lattice with negligible J ⊥ , cf . Fig. 2 . This suggests that the ab planes in TK91, which are separated by the CF 3 SO 3 − groups (see Fig. 1b ) are essentially decoupled. 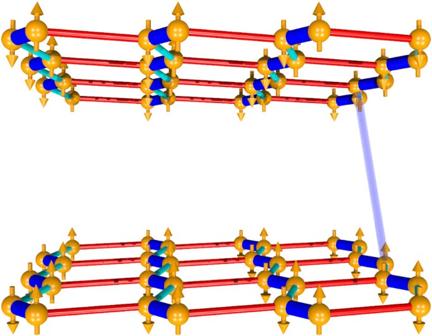Figure 2: Effective 2D dimer model of TK91. TheS=1/2 spins (arrows) at the copper ions (orange spheres) are antiferromagnetically coupled via moderately strongintra-dimerJd(dark-blue rods) and much weakerinter-dimer interactionsJ1(cyan rods) andJ2(red rods) within the (ab) planes. Adjacent layers are basically decoupled, that is,J⊥, indicated exemplarily by the glassy rod which corresponds to the Cu–Cu distanced3Cu–Cu=13.78 Å in the real structure inFig. 1, is zero within the accuracy of our DFT calculations. The interaction network has the topology of a 2D distorted honeycomb lattice. Figure 2: Effective 2D dimer model of TK91. The S =1/2 spins (arrows) at the copper ions (orange spheres) are antiferromagnetically coupled via moderately strong intra -dimer J d (dark-blue rods) and much weaker inter -dimer interactions J 1 (cyan rods) and J 2 (red rods) within the ( ab ) planes. Adjacent layers are basically decoupled, that is, J ⊥ , indicated exemplarily by the glassy rod which corresponds to the Cu–Cu distance d 3 Cu–Cu =13.78 Å in the real structure in Fig. 1 , is zero within the accuracy of our DFT calculations. The interaction network has the topology of a 2D distorted honeycomb lattice. Full size image Owing to the pronounced hierarchy in the exchange coupling constants, the dominant intra -dimer exchange interaction J d can be readily determined by thermodynamic probes [31] , [35] at high enough temperatures k B T>J 1 , J 2 , J ⊥ , where the system is expected to behave as an ensemble of independent dimers characterized by J d . In fact, the model of independent dimers for J d / k B =(9.5±0.2) K provides an excellent fit to the magnetic susceptibility and the specific heat for zero and moderately strong magnetic fields [31] , [35] and not too low temperatures (see Supplementary Fig. 1 and Supplementary Methods ). This confirms the independent-dimer character of TK91 for T >2 K and makes clear that all inter -dimer couplings must be significantly smaller. We stress that the experimentally determined J d is in remarkable agreement with the results of our DFT total energy calculations. Magnetic signatures of the field-induced triplon gas Given that the in-plane couplings J 1 , J 2 exceed any inter -layer coupling J ⊥ by at least one order of magnitude, as suggested by the DFT results, the application of a magnetic field, strong enough to close the dimer gap, is expected to give rise to a (quasi-) 2D gas of triplons, in analogy to the 3D case [4] . To explore the magnetic properties of this field-induced triplon gas, especially for disclosing potential field-induced ordering phenomena, high-resolution magnetic susceptibility and specific heat measurements have been performed at low temperatures extending down to k B T ≪ J 1 , J 2 . In Fig. 3 we show a selection of ac -susceptibility data as a function of magnetic field χ(H) =∂ M/ ∂ H for 5.5 T≤ μ 0 H ≤7.0 T. For fields outside this range up to the maximum field of 11 T accessible by our experiment, χ(H) ≈0, reflecting a constant magnetization M ( H ). Within the narrow field interval shown in Fig. 3 , χ(H) exhibits a pronounced structure the shape of which changes significantly with temperature. At T =281 mK ( Fig. 3a ), the χ ( H ) data reveal a single broadened peak centred at 6.2 T, reflecting singlet–triplet excitations of independent dimers. Upon cooling to below about 120 mK, however, the anomaly sharpens and a distinct double-peak structure develops. Upon further cooling to below 73 mK ( Fig. 3b,c ), the peaks become more pronounced. Most remarkably, however, even for the lowest temperature of 39 mK ( Fig. 3d ), the peaks remain distinctly rounded. We stress that an identical rounding was observed for all five single crystals investigated in the χ ( H ) experiments. 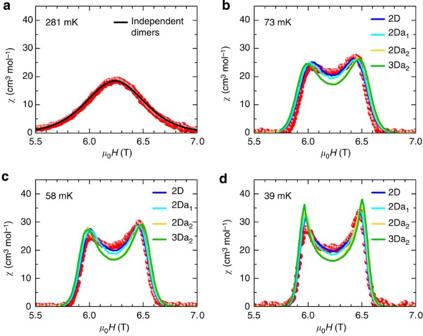Figure 3: Magnetic susceptibility as a function of the magnetic fieldμ0Hat varying temperatures. Red spheres represent magnetic susceptibility data taken on single-crystalline samples (crystal no. 5 inaand crystal no. 7 inb–d) of C36H48Cu2F6N8O12S2(TK91), see section Methods for the determination of the absolute values ofχ. Black solid line inacorresponds to singlet–triplet excitations of independent dimers. The solid lines inb–dare results of Quantum Monte Carlo simulations for the 2D distorted honeycomb lattice shown inFig. 2using anintra-dimer coupling ofJd/kB=9.507 K and three differentinter-dimer coupling schemes. Dark-blue line (2D): two-dimensionally coupled dimers withJ1/kB=J2/kB=J||/kB=0.325 K; cyan line (2Da1) and yellow line (2Da2): anisotropic two-dimensionally coupled dimers withJ1/kB=0.450 K,J2/kB=0.200 K andJ1/kB=0.550 K,J2/kB=0.100 K, respectively; green line (3Da2): anisotropic three-dimensionally coupled dimers withJ1/kB=0.55 K,J2/kB=0.1 K andJ⊥/kB=0.02 K. The statistical errors in the QMC data are of the order of the line width. Figure 3: Magnetic susceptibility as a function of the magnetic field μ 0 H at varying temperatures. Red spheres represent magnetic susceptibility data taken on single-crystalline samples (crystal no. 5 in a and crystal no. 7 in b – d ) of C 36 H 48 Cu 2 F 6 N 8 O 12 S 2 (TK91), see section Methods for the determination of the absolute values of χ . Black solid line in a corresponds to singlet–triplet excitations of independent dimers. The solid lines in b – d are results of Quantum Monte Carlo simulations for the 2D distorted honeycomb lattice shown in Fig. 2 using an intra -dimer coupling of J d /k B =9.507 K and three different inter -dimer coupling schemes. Dark-blue line (2D): two-dimensionally coupled dimers with J 1 /k B = J 2 /k B = J || /k B =0.325 K; cyan line (2Da 1 ) and yellow line (2Da 2 ): anisotropic two-dimensionally coupled dimers with J 1 /k B =0.450 K, J 2 /k B =0.200 K and J 1 /k B =0.550 K, J 2 /k B =0.100 K, respectively; green line (3Da 2 ): anisotropic three-dimensionally coupled dimers with J 1 /k B =0.55 K, J 2 /k B =0.1 K and J ⊥ /k B =0.02 K. The statistical errors in the QMC data are of the order of the line width. Full size image The double-peak structure in the low-temperature χ ( H ) data in Fig. 3 indicates the evolution of magnetization M ( H ) within a narrow field range. Integrating the χ ( H,T= 39 mK) data yields a saturation magnetization consistent with the high-field state being fully spin-polarized. Signatures in χ ( H,T= constant) at H c1 and H c2 , with H c1 denoting the critical field where the lower triplon branch crosses zero energy, and H c2 the field above which all dimers are fully polarized, are also expected and found in 3D-coupled systems [36] . Unlike these 3D systems, however, where sharp, λ -like peaks in thermodynamic quantities indicate thermodynamic transitions at the on- and off-set of conventional long-range order [37] , [38] no indications of such λ-like peaks are revealed in χ ( H, T= constant) for TK91. These isothermal χ ( H ) measurements were supplemented by temperature-dependent measurements in a constant field of both the magnetic susceptibility χ ( T, H= constant) as well as the specific heat C ( T, H= constant). Although for the magnetic part of the specific heat C mag larger uncertainties have to be accepted, as compared with χ , because of substantial nuclear and nonmagnetic contributions (see Supplementary Fig. 2 and Supplementary Methods ), C ( T ) may provide important additional information. It allows for tracking a potential phase transition and also enables a consistency check to be performed for the model parameters derived from analysing the χ ( H ) data. In Fig. 4 we show the low-temperature susceptibility and magnetic specific heat C mag both taken at the same field value of μ 0 H =6.23 T≈ μ 0 ( H c1 + H c2 )/2. The C mag data reveal a broad maximum around 120 mK, indicative of 2D magnetic correlations (see, for example, refs 39 , 40 , 41 , 42 ), followed by a rounded peak near 50 mK. To check whether or not the latter effect is because of an inhomogeneously broadened magnetic transition, the figure also shows χ ( T, H= 6.23 T) data for the same temperature range. Beside a broad maximum centred at 150 mK, reflecting the 2D magnetic character, the data lack any indication for a phase transition down to 27 mK, the lowest temperature accessible by this experiment. This rules out a magnetic transition as the origin for the peak in C mag around 50 mK even if allowing for considerable inhomogeneous broadening, for which indications were found neither in the magnetic measurements ( Fig. 3 ) nor in thorough structural characterization measurements on various TK91 crystals studied in this work. Instead, as will be shown below, a broadened peak in C (and C / T ) is, in fact, a feature expected for 2D systems. 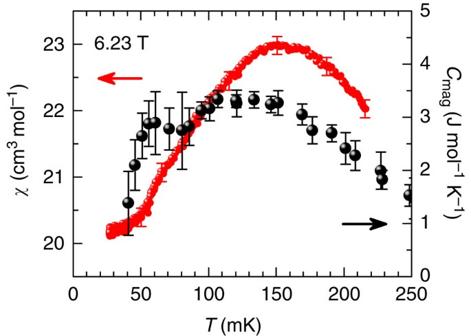Figure 4: Experimental data of the magnetic specific heat and the magnetic susceptibility as a function of temperature. Black and red spheres show on the same temperature axis results of the magnetic specific heat (right scale) and the magnetic susceptibility (left scale), respectively, of the spin dimers of single-crystalline C36H48Cu2F6N8O12S2(TK91) at a field ofμ0H=6.23 T applied parallel to theaaxis. For the determination of the absolute values ofχ, see section Methods. Figure 4: Experimental data of the magnetic specific heat and the magnetic susceptibility as a function of temperature. Black and red spheres show on the same temperature axis results of the magnetic specific heat (right scale) and the magnetic susceptibility (left scale), respectively, of the spin dimers of single-crystalline C 36 H 48 Cu 2 F 6 N 8 O 12 S 2 (TK91) at a field of μ 0 H =6.23 T applied parallel to the a axis. For the determination of the absolute values of χ , see section Methods. Full size image QMC modelling For a detailed understanding of the anomalies observed in χ ( H ) and C mag ( T ) at lowest temperatures T ≤150 mK, especially with regard to the dimensionality of the interactions and the implications for the type of order that is realized here, QMC simulations have been performed. On the basis of the low-energy spin-lattice geometry obtained from DFT calculations, we assume a general form of a spin-1/2 Heisenberg model on an anisotropic honeycomb lattice as shown in Fig. 2 . QMC simulations were performed for models with different anisotropies in the magnetic couplings, also including the effect of a finite inter -plane coupling J ⊥ . The range and possible combinations of exchange parameters to be considered in the analysis are constrained by the positions of the low- and high-field peaks in χ(H) , cf . Fig. 3b–d . By assigning the latter with H c1 and H c2 , respectively, and assuming a dominant intra -dimer exchange J d , the effective spin exchange parameters can be estimated from an expansion of H c1 and H c2 up to first order in the inter -dimer exchange. For the present geometry this yields gμ B μ 0 H c1 = J d − ( J 1 + J 2 + J ⊥ )/2 and gμ B μ 0 H c2 = J d + J 1 + J 2 + J ⊥ . Note that the latter formula is exact as H c2 equals the saturation field. Using μ 0 H c1 =5.909 T and μ 0 H c2 =6.55 T, as taken from Fig. 3 for T =39 mK, and for g =2.309, yields J d /k B =9.507 K and J 1 /k B + J 2 /k B =0.65 K for strictly 2D models ( J ⊥ =0). Note that ESR experiments reveal a slightly smaller g -value of 2.27 at 108 K [31] . The small increase in g of Δ g =0.04 is attributed to temperature-induced changes of the local Cu-coordination sphere upon cooling from 108 K down to sub-Kelvin temperatures. To study the effect of a weak inter -layer coupling J ⊥ , still compatible with the DFT calculations, we set J ⊥ /k B =0.02 K while keeping J 1 /k B + J 2 /k B =0.65 K. In the following, we will use the QMC simulations for various coupling schemes to derive model parameters that provide a good description of the magnetic susceptibility data in Fig. 3 . In a second step, we will then check the so-derived parameters for consistency with the C mag ( T ) data in Fig. 4 . As Fig. 3 demonstrates the anisotropic 3D model (labelled 3Da 2 ) does not describe the data well, especially it deviates significantly from the data around the peaks and the minimum. Note that the latter effect is a consequence of the strong in-plane anisotropy of this model. The model description becomes considerably improved, however, by waiving the inter -layer coupling, that is, by considering purely 2D models. While the isotropic (2D) and moderately anisotropic (2Da 1 ) models fit the data almost equally well, the strongly anisotropic variant (2Da 2 ) deviates from the data substantially. As indicated in Fig. 3b,c , the 2D and 2Da 1 models with the same parameters, as used in Fig. 3d , also provide a good description of the double-peak structure upon increasing the temperature to 58 and 73 mK. The same set of parameters is also used for QMC simulations of C mag ( T, H= const), plotted as C mag / T in Fig. 5 to emphasize the interesting low-temperature part of the data more clearly. Consistent with the simulations shown in Fig. 3 for χ (H,T=const), the 2D models are found to qualitatively reproduce the characteristic features of C mag ( T )/ T , including the gradual growth upon cooling and the broad peak at low temperatures. The simulations yield such a peak for the isotropic case (2D), although more strongly pronounced and at somewhat higher temperatures as compared with the experimental data. By introducing an anisotropy in the model, the peak becomes significantly reduced in size and shifted to lower temperatures with increasing anisotropy, that is, by going to the 2Da 1 and the 2Da 2 models. Quantitatively, taking the experimental uncertainties into account, the data in Fig. 5 are consistent with the anisotropic 2Da 1 and 2Da 2 models but incompatible with the isotropic 2D variant. To study the effect of a weak inter -layer coupling, we exemplarily show QMC simulations for the 3Da 2 model. The simulations indicate that by turning on J ⊥ the broad maximum of the 2Da 2 model shifts to higher temperatures, grows significantly in size and sharpens. We assign this feature to the phase transition into long-range magnetic order as expected for a 3D-coupled system. 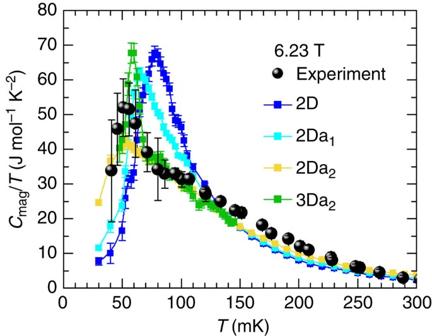Figure 5: Magnetic specific heat divided by temperature as a function of temperature. Large black spheres represent results of the magnetic specific heat in a representationCmag/T.Cmaghas been derived from the measured specific heat by subtracting the nuclear contribution resulting from the protons (1H), copper (63Cu and65Cu) and fluorine (19F) nuclei, contained in TK91 according to their natural abundances, and a Schottky-like anomaly centred around 0.4 K. Since the latter feature is independent of magnetic fields for 4 T≤μ0H≤8 T, it is likely of structural origin (seeSupplementary Figs 2 and 3). Note that the subtraction of these contributions, which can be well accounted for by smooth analytical functions (Schottky anomalies), implies some uncertainties in the overall shape and absolute values of the so-derivedCmag(T, H=constant) data. However, this procedure does not affect the fine structure inCmag(T)/T, especially the broad peak around 50 mK. Enhanced error bars at low temperatures are because of the enhanced relaxation times as a consequence of the large total specific heat (seeSupplementary Fig. 2). The small symbols connected by thin lines are the results of QMC simulations for the same model parameters as shown inFig. 3. Dark-blue squares (2D): two-dimensionally coupled dimers withJ1/kB=J2/kB=J||/kB=0.325 K; cyan squares (2Da1) and yellow squares (2Da2): anisotropic two-dimensionally coupled dimers withJ1/kB=0.450 K,J2/kB=0.200 K andJ1/kB=0.550 K,J2/kB=0.100 K, respectively. Green squares (3Da2): anisotropic three-dimensionally coupled dimers withJ1/kB=0.55 K,J2/kB=0.1 K andJ⊥/kB=0.02 K to study the effect of introducing a smallinter-layer couplingJ⊥to the parameters of the 2Da2model. The same trend, that is, the emergence of a sharp peak on the high-temperature flank of the maximum revealed in the simulations for the corresponding anisotropic 2D model, is seen also for the 3Da1model withJ1/kB=0.450 K,J2/kB=0.200 K andJ⊥/kB=0.02 K (seeSupplementary Fig. 4), yielding a pronounced and sharp maximum around 75 mK, clearly incompatible with the experimental data. Figure 5: Magnetic specific heat divided by temperature as a function of temperature. Large black spheres represent results of the magnetic specific heat in a representation C mag / T . C mag has been derived from the measured specific heat by subtracting the nuclear contribution resulting from the protons ( 1 H), copper ( 63 Cu and 65 Cu) and fluorine ( 19 F) nuclei, contained in TK91 according to their natural abundances, and a Schottky-like anomaly centred around 0.4 K. Since the latter feature is independent of magnetic fields for 4 T≤ μ 0 H ≤8 T, it is likely of structural origin (see Supplementary Figs 2 and 3 ). Note that the subtraction of these contributions, which can be well accounted for by smooth analytical functions (Schottky anomalies), implies some uncertainties in the overall shape and absolute values of the so-derived C mag ( T, H= constant) data. However, this procedure does not affect the fine structure in C mag ( T )/ T , especially the broad peak around 50 mK. Enhanced error bars at low temperatures are because of the enhanced relaxation times as a consequence of the large total specific heat (see Supplementary Fig. 2 ). The small symbols connected by thin lines are the results of QMC simulations for the same model parameters as shown in Fig. 3 . Dark-blue squares (2D): two-dimensionally coupled dimers with J 1 /k B = J 2 /k B = J || /k B =0.325 K; cyan squares (2Da 1 ) and yellow squares (2Da 2 ): anisotropic two-dimensionally coupled dimers with J 1 /k B =0.450 K, J 2 /k B =0.200 K and J 1 /k B =0.550 K, J 2 /k B =0.100 K, respectively. Green squares (3Da 2 ): anisotropic three-dimensionally coupled dimers with J 1 /k B =0.55 K, J 2 /k B =0.1 K and J ⊥ /k B =0.02 K to study the effect of introducing a small inter -layer coupling J ⊥ to the parameters of the 2Da 2 model. The same trend, that is, the emergence of a sharp peak on the high-temperature flank of the maximum revealed in the simulations for the corresponding anisotropic 2D model, is seen also for the 3Da 1 model with J 1 /k B =0.450 K, J 2 /k B =0.200 K and J ⊥ /k B =0.02 K (see Supplementary Fig. 4 ), yielding a pronounced and sharp maximum around 75 mK, clearly incompatible with the experimental data. Full size image Taken together, the good agreement of the QMC simulations for the 2Da 1 model with the magnetic susceptibility and the consistency with the specific heat demonstrate that an anisotropic, purely 2D Heisenberg model of weakly interacting dimers provides a suitable basis for describing the field-induced effects observed in TK91 at low temperatures. The 2D character implies that the state realized here cannot be ascribed to the usual field-induced long-range antiferromagnetism, tantamount to BEC of triplons, but has to be assigned to a collectively coupled-dimer state of distinctly different type. In fact, as pointed out by Berezinskii, Kosterlitz and Thouless [11] , [12] , [13] , a different scenario, involving vortices as topologically stable excitations, driving a phase transition associated with topological order at a temperature T BKT , is inherent to the 2D XY model. This raises the question whether the 2D XY model is applicable to the anomalous state encountered in TK91 for H c1 ≤ H ≤ H c2 . Indeed, as pointed out by various authors [41] , [43] , a BKT transition and generic XY behaviour can be found also in an S =1/2 2D Heisenberg antiferromagnet by the application of a finite magnetic field along the z axis, which breaks the O (3) symmetry of the isotropic model. We stress that for dimerized systems such as TK91, which are gapped for H < H c1 , this scenario is applicable for H c1 < H < H c2 as the low-energy physics can be mapped on an effective easy-plane spin-1/2 XXZ model at a field H — H c1 (ref. 44 ). In order to identify the field and temperature range where the topological order is expected to be stabilized in TK91, we perform QMC calculations for the parameters of the 2Da 1 model to estimate the helicity modulus Y . Here Y is obtained from the spin-winding numbers in the QMC simulations [45] . The BKT transition is then given by the temperature/field values at which Y crosses the universal line Y =2 T / π (see, for example, ref. 46 ). As an example, we show in Fig. 6 (upper panel) Y at a constant field μ 0 H =6.144 T as a function of temperature. This field value is close to the middle between H c1 and H c2 where T BKT is expected to be maximal. 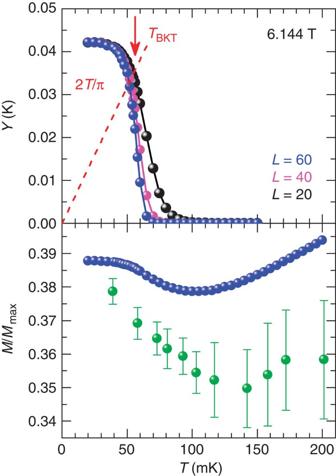Figure 6: Helicity modulus and uniform magnetization. Upper panel: QMC results of the helicity modulus for the anisotropic 2D dimer model (2Da1) for systems of linear sizeLas a function of temperature in a magnetic fieldμ0H=6.144 T. The calculations are based on the same parameters as used for the 2Da1curves inFig. 3. The broken straight line corresponds to the universal curve 2T/π,and the arrow marks the transition temperatureTBKTobtained from the finite-size analysis as mentioned in the main text. The BKT topological order is stable in the temperature and field range whereY≥2T/π. In order to extract the BKT transition temperature from the finite-size data, we employed an analysis following Weber and Minnhagen56(see also ref.57for the quantum case), based on the finite-size scaling formπY/(2T)=A(T)·(1+1/(2log[L/L0(T)])), whereLdenotes the linear system size andL0a fitting parameter, and which is correct at the transition point withA(TBKT)=1. Lower panel: normalized magnetization derived from QMC calculations (blue spheres) with the same parameters as used in the upper panel and by integrating experimentalχ(H,T=constant) curves (green spheres).Mmaxcorresponds to the magnetization of the fully polarized state atH>Hc2. The experimental data (green spheres) have been shifted by +0.015 (corresponding to 4%). This offset inMcorresponds to the difference in the areas under theχ(H,T=39 mK) data and the 2Da1QMC results inFig. 3d. The minimum in the magnetization well aboveTBKTrevealed for both data sets signals the crossover from isotropic behaviour at higher temperatures to low-T XYbehaviour. The statistical errors in the QMC data in the upper and lower panels are below symbol size. Figure 6: Helicity modulus and uniform magnetization. Upper panel: QMC results of the helicity modulus for the anisotropic 2D dimer model (2Da 1 ) for systems of linear size L as a function of temperature in a magnetic field μ 0 H =6.144 T. The calculations are based on the same parameters as used for the 2Da 1 curves in Fig. 3 . The broken straight line corresponds to the universal curve 2 T/π, and the arrow marks the transition temperature T BKT obtained from the finite-size analysis as mentioned in the main text. The BKT topological order is stable in the temperature and field range where Y ≥2 T / π . In order to extract the BKT transition temperature from the finite-size data, we employed an analysis following Weber and Minnhagen [56] (see also ref. 57 for the quantum case), based on the finite-size scaling form πY /(2 T ) =A ( T )·(1+1/(2log[ L/L 0 ( T )])), where L denotes the linear system size and L 0 a fitting parameter, and which is correct at the transition point with A ( T BKT )=1. Lower panel: normalized magnetization derived from QMC calculations (blue spheres) with the same parameters as used in the upper panel and by integrating experimental χ ( H,T= constant) curves (green spheres). M max corresponds to the magnetization of the fully polarized state at H > H c2 . The experimental data (green spheres) have been shifted by +0.015 (corresponding to 4%). This offset in M corresponds to the difference in the areas under the χ ( H,T= 39 mK) data and the 2Da 1 QMC results in Fig. 3d . The minimum in the magnetization well above T BKT revealed for both data sets signals the crossover from isotropic behaviour at higher temperatures to low- T XY behaviour. The statistical errors in the QMC data in the upper and lower panels are below symbol size. Full size image The results of these QMC calculations, compiled in Fig. 7 , indicate that a BKT topological order is expected in TK91 in magnetic fields 5.95 T≤ μ 0 H ≤6.5 T with a maximum BKT transition temperature of ~50 mK obtained in a field of 6.2 T. Comparative calculations for the isotropic 2D model, yielding virtually the same stability range of the BKT order, indicate that in-plane ( J 1 , J 2 ) anisotropies have only little effect on the BKT phase. For comparison, Fig. 7 also includes the positions of the χ ( H,T= const) maxima as read off the data in Fig. 3b–d , which define the range of stability of the 2D collectively coupled-dimer state. Within the effective easy-plane XXZ model description of the 2D coupled-dimer system, the onset of this region (blue area in Fig. 7 ) can be assigned to the crossover from the high- T isotropic to the low- T XY behaviour of the effective spins, which also marks the onset of the formation of vortices and antivortices emerging in the effective spin configurations. This assignment is corroborated by exploring the uniform magnetization M(T) at a constant field μ 0 H =6.144 T. To this end, we compare in the lower panel of Fig. 6 M(T) results of our QMC calculations with experimental data obtained by integrating the various χ ( H,T= const) curves from 5.5 to 6.144 T. Both data sets reveal a distinct minimum at a temperature T min considerably above T BKT . As has been discussed in ref. 38 for a square-lattice configuration, the growth in the magnetization for T BKT < T < T min is a clear signature of the crossover to XY behaviour. Note that at T BKT no anomaly is expected in M ( T ) and C ( T ), as the BKT transition does not involve any spontaneous symmetry breaking, consistent with the experimental results. 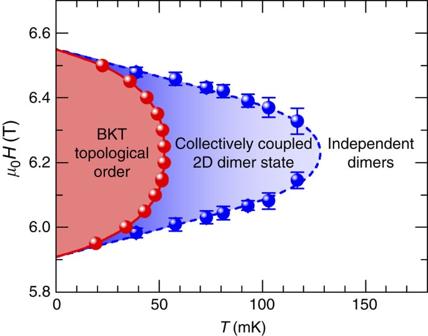Figure 7: Magnetic field versus temperature diagram of TK91. The red symbols mark points where QMC calculations of the helicity modulus for the anisotropic 2D model (2Da1) indicate the transition into the BKT phase. The statistical errors are below symbol size. The red solid line, delimiting the stability range of the BKT phase (red area), is a guide for the eyes. The blue symbols give the positions of the maxima in the susceptibility as derived from experimentalχ(H,T=constant) data taken at varying temperatures. With increasing temperatures the maxima become blurred,cf.Fig. 3, and are no longer discernable above 120 mK. The blue area marks the crossover range where the behaviour changes fromisotropicoutside (white area) toXYbehaviour accompanied by the formation of vortices and antivortices in the effective spin configurations. Figure 7: Magnetic field versus temperature diagram of TK91. The red symbols mark points where QMC calculations of the helicity modulus for the anisotropic 2D model (2Da 1 ) indicate the transition into the BKT phase. The statistical errors are below symbol size. The red solid line, delimiting the stability range of the BKT phase (red area), is a guide for the eyes. The blue symbols give the positions of the maxima in the susceptibility as derived from experimental χ ( H,T= constant) data taken at varying temperatures. With increasing temperatures the maxima become blurred, cf . Fig. 3 , and are no longer discernable above 120 mK. The blue area marks the crossover range where the behaviour changes from isotropic outside (white area) to XY behaviour accompanied by the formation of vortices and antivortices in the effective spin configurations. Full size image Figure 7 indicates that the on- and offset fields of this crossover range merge with the corresponding fields that delimit the BKT topological order for T →0. We therefore conclude that the novel field-induced state, clearly revealed by the isothermal susceptibility measurements at the lowest temperature of our experiment of 39 mK, is likely a manifestation of the BKT topological order, which is preceded on the temperature axis by a range (blue area in Fig. 7 ) governed by vortex excitations. It has been argued [43] , [47] that a finite inter -plane coupling J ⊥ should lead to true 3D long-range order below a Néel temperature T N > T BKT . In TK91, however, the ab planes appear essentially decoupled, at least when compared with the expected anisotropic 3D behaviour for J ⊥ / k B =0.02 K studied in our QMC simulations, and consistent with the results of temperature-dependent susceptibility measurements, setting an upper limit for a potential Néel ordering of T N <27 mK. We believe that this dimensional reduction in TK91 is a consequence of the simultaneous action of several of such very weak inter -plane interactions that compensate each other due to frustration. One possible experimental route to directly probe the emergence of BKT physics in TK91 would be to perform neutron-scattering experiments on sufficiently large single crystals. Although at this point these crystals are not available, we provide here theoretical predictions for the magnetic structure factor that relates to the neutron-scattering intensity. For this purpose, we show in Fig. 8 the transverse spin structure factor S ( q )=½‹ S + ( q ) S − ( q )+ h.c. ›, the Fourier transform of the transverse spin–spin correlations, for different temperatures as a function of the transfer momentum q =( q x , q y ,0) taken parallel to the 2D dimer layers of TK91. While at 200 mK ( Fig. 8c ) only mild variations in S ( q ) are visible, at 70 mK, that is, within the collectively coupled 2D dimer state ( cf . Fig. 7 ), the emerging peak structure is already well developed. The peak heights increase strongly upon further approaching the BKT transition temperature. The detection of the peak signals upon cooling the sample should thus allow for an identification of the collectively coupled regime via neutron-scattering experiments. Such temperature-dependent measurements, together with the demonstration that the scattering intensity is independent of q z , the component of the transfer momentum perpendicular to the 2D dimer layers, would provide a direct experimental test of BKT physics in TK91. 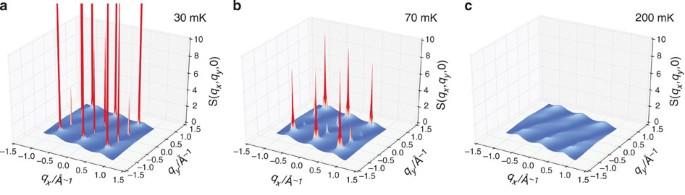Figure 8: Calculated transversal structure factor of TK91. The data are the results of QMC simulations for TK91 on a lattice with 48 × 48 sites using the in-plane magnetic exchange couplings for the anisotropic 2D model (2Da1). The calculations were performed for a fieldμ0H=6.23 T and temperatures of 30 (a), 70 (b) and 200 mK (c). The overall magnetic signal is finite-size-converged, apart from the peak heights at 30 mK (a), which diverge in the infinite system limit, whileS(q)/N, withNthe number of spins, vanishes in the thermodynamic limitN→∞, in accord with the absence of true long-range order. At 70 mK one can also clearly identify a modulation in the peak heights that results from the fact that more than one magnetic moment resides within the lattice unit cell. The finite deviation of the peak positions with respect toq=0 relates to the dominant antiferromagnetic coupling within the 2D planes; in a state with true long-range order, these peak positions correspond to the doubling of the unit cell from the antiferromagnetic transverse order. Figure 8: Calculated transversal structure factor of TK91. The data are the results of QMC simulations for TK91 on a lattice with 48 × 48 sites using the in-plane magnetic exchange couplings for the anisotropic 2D model (2Da 1 ). The calculations were performed for a field μ 0 H =6.23 T and temperatures of 30 ( a ), 70 ( b ) and 200 mK ( c ). The overall magnetic signal is finite-size-converged, apart from the peak heights at 30 mK ( a ), which diverge in the infinite system limit, while S ( q )/ N , with N the number of spins, vanishes in the thermodynamic limit N →∞, in accord with the absence of true long-range order. At 70 mK one can also clearly identify a modulation in the peak heights that results from the fact that more than one magnetic moment resides within the lattice unit cell. The finite deviation of the peak positions with respect to q =0 relates to the dominant antiferromagnetic coupling within the 2D planes; in a state with true long-range order, these peak positions correspond to the doubling of the unit cell from the antiferromagnetic transverse order. Full size image In summary, by assembling Cu ( S =1/2)-based dinuclear building blocks (dimers), we were able to generate a chemically constructed multilayer magnet that lacks long-range 3D magnetic order down to 27 mK, the lowest temperature of our experiment. Elaborate ab initio DFT calculations indicate that the low-energy properties of the material can be described by an effective quasi-2D dimer model on a distorted honeycomb lattice with moderately strong in-plane anisotropy. The hierarchy in the hopping integrals derived from these calculations, together with a dominant intra -dimer exchange coupling J d /k B of about 9.5 K, as determined from thermodynamic studies, imply that for temperatures k B T < J d the application of a moderate field will induce a gas of mobile triplon excitations. By employing high-resolution susceptibility and specific heat measurements combined with QMC simulations, we show that these excitations have a distinct 2D character. This implies an extended magnetic field and temperature range where vortex excitations prevail followed by a low-temperature state, revealed at 39 mK, which is likely a manifestation of the topological order predicted by Berezinskii, Kosterlitz and Thouless. Experiment The susceptibility data shown in Figs 3 and 6 were recorded by using an ultrahigh resolution ac-susceptometer adapted to a 3 He– 4 He dilution refrigerator. The compensated-coil susceptometer is size-optimized for measuring the small single crystals of TK91. The amplitude of the applied ac-field was μ 0 H ac =0.9 mT (0.5 mT) at a frequency of f =16 Hz (81 Hz) for the data shown in Figs 3 and 6 . The sweep-rate of the external dc-field μ 0 H was set below 0.2 mT s −1 giving rise to an induced dc-signal that is three orders of magnitude smaller than the sample signal. The magnetic field has been applied along the needle axis ( a axis) of the small single crystals, the mass of which ranges from 0.1 to 0.2 mg. The sample temperature during the field sweeps was stabilized within ±0.2 mK. Consecutive runs for the same settings give reproducible results with maximum deviations of ~2%. The susceptibility values have all been multiplied by the same factor, chosen in such a way that for 39 mK the magnetic field integral of the susceptibility between 5.5 and 7.0 T yields the same value as for the theory curve. By this procedure we account for uncertainties in the experimental data resulting from uncertainties in the sample mass, the geometry factor of the secondary coil and the demagnetization factor of the sample. The specific heat measurements were conducted by using a high-resolution (Δ C ≥25 nJ K −1 ) relaxation calorimeter adapted to a 3 He– 4 He dilution refrigerator on two single crystals with masses of 2.08 and 0.10 mg. A magnetic field of μ 0 H =6.23 T was applied along the needle axis ( a axis). To reduce statistical errors, individual data points represent the average over several independent measurements. The change Δ T of the sample temperature, after changing the applied heating power in the used relaxation technique, was kept below 2% of the sample temperature T except for T <100 mK. In this range, Δ T was chosen such that Δ T / T gradually increases reaching 4.5% at 40 mK. Theory The ab initio DFT calculations involve a combination of the linear augmented plane wave method [48] and the NMTO method [33] . Results were cross-checked among the two schemes in terms of energy differences, density of states and band structure. We considered as exchange-correlation functionals the generalized-gradient approximation (GGA) and the LSDA+ U scheme [49] . The so-derived band structure for TK91 in the triclinic crystal symmetry within GGA shows the formation of two narrow bands crossing the Fermi energy. These bands correspond to the two Cu ions in the unit cell and are predominantly of Cu d x 2 − y 2 character. They are separated from the rest of the valence bands of O -p , F -p , C -p , H -s and Cu d , d xy , d xz , d yz character by a gap of ~0.8 eV. The bands crossing the Fermi energy are half-filled. Therefore, the inclusion of correlation effects beyond GGA, as implemented in the LSDA+ U functional, drives the system to an (Mott) insulating state. In order to derive a low-energy, few-band Hamiltonian from the full band structure, we have applied the NMTO-downfolding procedure [33] . By this method a low-energy Hamiltonian is derived by considering the Löwdin partitioning technique [34] which integrates out high-energy states after partitioning the Hilbert space of the full system into states of interest (low-energy bands) and high-energy bands. The low-energy Hamiltonian is then defined in the basis of effective Wannier-like orbitals and its real-space representation H =∑ ij t ij ( c i + c j + h.c .) in the Wannier function basis gives the various hopping integrals t ij between the effective orbitals. Our total energy calculations were performed with the Full Potential Local Orbital code [50] within the LSDA+ U scheme [51] . We considered supercells of TK91 of various sizes with different Cu-spin configurations. Up to 18 k -points in the irreducible part of the Brillouin zone were used. Total energy differences were then mapped to a spin-1/2 Heisenberg model [52] . From the total energy calculations, the error bars in the J / k B values, being typically of the order of 0.1–1 K, can be estimated by considering the combined uncertainties arising from the finite k -mesh and the freedom of choosing different spin configurations for the determination of the exchange constants. For the QMC calculations, the stochastic series expansion algorithm [53] was used, employing a generalized directed loop update [54] , [55] . The finite-temperature simulations are performed on lattices with up to 80 × 80 spins for the purely 2D case, and up to 40 3 lattice sites for the quasi-3D simulations. Except for the helicity modulus, we find that within the considered temperature range the results are size-converged within error bars for system sizes beyond 60 × 60 in 2D, and 30 3 for the quasi-3D case. How to cite this article: Tutsch, U. et al. Evidence of a field-induced Berezinskii–Kosterlitz–Thouless scenario in a two-dimensional spin–dimer system. Nat. Commun. 5:5169 doi: 10.1038/ncomms6169 (2014).